Pitfalls in using phenanthroline to study the causal relationship between promoter nucleosome acetylation and transcription 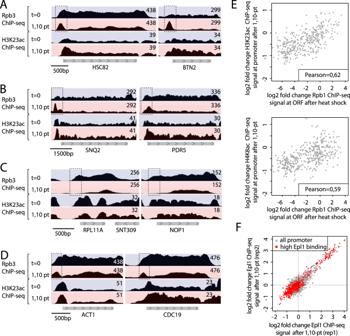Fig. 1: 1,10-pt induces a stress response affecting RNAPII and Epl1 promoter binding. A–DGenome browser tracks showing RNAPII (Rpb3) or H3K23 acetylation ChIP-seq read counts at the indicated genes before (t= 0) or 15 min after 1,10-pt treatment. Dashed boxes indicate promoter regions where Rpb3 binding either decreases or increases (possibly in an elongation-block state) following 1,10-pt treatment. Raw data are from Martin et al.1.EScatter plot comparing H3K23ac (top) and H4K8ac (bottom) at promoters 15 min following 1,10-pt treatment (y-axis) to Rpb1 ChIP-seq (all fold-change, log2) at 5 min following heat shock (x-axis) for the 400 most highly expressed genes. Pearson coefficient is indicated. Raw data are from Martin et al.1for H3K23ac and H4K8ac ChIP-seq and13for Rpb1 ChIP-seq.FScatter plot comparing two replicates (Rep1 and Rep2) measuring log2 fold change of Epl1 ChIP-seq signal before and after 1,10-pt treatment at all RNAPII promoters (gray dots) or at 562 promoters displaying high Epl1 binding in the absence of 1,10-pt (red dots), selected by Martin et al.1. Raw data are from ref.1. 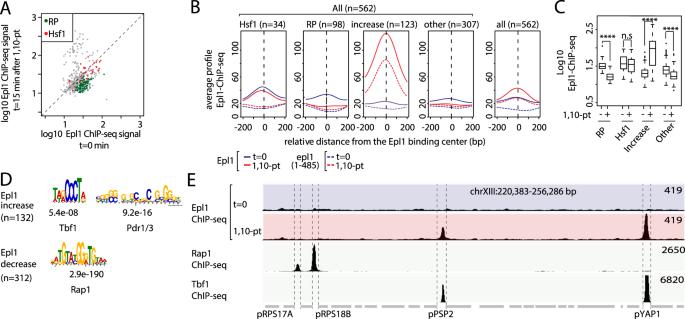Fig. 2: 1,10-pt treatment mostly leads to a significant decrease in Epl1 promoter binding except for a small group of genes displaying a dramatic Epl1 binding increase. AScatter plots comparing Epl1 ChIP-seq signal before and after 1,10-pt treatment at promoters of all 562 genes (gray dots) selected by Martin et al.1to study Epl1 promoter binding. Indicated gene categories (RP genes,n= 98; Hsf1 target genes,n= 34) are color-coded on the scatter plots; raw data are from replicate 1 from ref.1.BAverage Epl1 or Epl1(1-485) (dotted line) binding profiles on genes selected by Martin et al.1) before (blue curves) or after 15 min of 1,10-pt treatment (red curves). The first four panels show data for all 562 genes divided into four separate categories, as marked: Hsf1 target genes (Hsf1,n= 34), ribosomal protein genes (RP,n= 98), genes where Epl1 ChIP-seq signal increases > 1,2 fold (Increase,n= 123), and all other genes in this group (Other,n= 307). The right-most panel shows the average for all 562 genes. Data are taken from Martin et al.1and all plots are centered on the Epl1 signal peak.CBoxplots of log10 EpL1 ChIP-seq signal at promoters of the four gene categories defined inBbefore (−) or after (+) 15 min of 1,10-pt treatment. The ChIP-seq signal is quantified in a region delimited as the 100 bp region upstream and downstream of the Epl1 signal peak defined by Martin et al.1. Asterisks show significant difference according to the Wilcoxon test (*P< 0.05, **P< 0.01, ***P< 0.001, ns not significant).DMost significant motifs found in genes at which Epl1 binding increases (>1,2-fold) or decreases (<0,8-fold) after 1,10-pt treatment. E values and the TF associated with the consensus binding motif identified by MEME are indicated.EGenome browser tracks showing Epl1, Rap1 and Tbf1 ChIP-seq read counts at the promoter regions (roughly demarcated by dotted lines) of the indicated genes before (t= 0) or 15 min after 1,10-pt treatment. Raw data are from Martin et al.1, Knight et al.17, and Preti et al.18and for Epl1, Rap1, and Tbf1 ChIP-seq, respectively. Data analysis ChIP-seq datasets (Replicate 1) from 1,10-pt-treated or untreated cells were normalized to silent regions by ChIP Normalization Factors calculated in ref. [1] . ChIP-seq signal was quantified for each promoter defined as the 400 bp region upstream of the transcription start site (TSS), as obtained from ref. [15] . To calculate ChIP-seq signals fold change, a ratio between the total number of reads for each promoter from 1,10-pt treated cells and the number of reads from untreated cells was made. RP gene list was defined in ref. [14] and Hsf1 gene list in ref. [7] . Statistics Yeast Mine ( https://yeastmine.yeastgenome.org/yeastmine/begin.do ) was used to determine GO-terms and MEME [16] was used for motif enrichment analysis, with the following settings: anr -nmotifs 5 -minw 6 -maxw 20 -objfun classic -revcomp -markov_order 0. In all of the box plots, the box shows the 25th–75th percentile, whiskers show the 10th–90th percentile, and dots show the 5th and 95th percentiles. Asterisks show significant difference according to the Wilcoxon test (* P < 0.05, ** P < 0.01, *** P < 0.001, ns not significant). Reporting summary Further information on research design is available in the Nature Research Reporting Summary linked to this article.